Hydrogenosomes in the diplomonadSpironucleus salmonicida Acquisition of the mitochondrion is a key event in the evolution of the eukaryotic cell, but diversification of the organelle has occurred during eukaryotic evolution. One example of such mitochondria-related organelles (MROs) are hydrogenosomes, which produce ATP by substrate-level phosphorylation with hydrogen as a byproduct. The diplomonad parasite Giardia intestinalis harbours mitosomes, another type of MRO. Here we identify MROs in the salmon parasite Spironucleus salmonicida with similar protein import and Fe–S cluster assembly machineries as in Giardia mitosomes. We find that hydrogen production is prevalent in the diplomonad genus Spironucleus , and that S. salmonicida MROs contain enzymes characteristic of hydrogenosomes. Evolutionary analyses of known hydrogenosomal components indicate their presence in the diplomonad ancestor, and subsequent loss in Giardia . Our results suggest that hydrogenosomes are metabolic adaptations predating the split between parabasalids and diplomonads, which is deeper than the split between animals and fungi in the eukaryotic tree. All extant eukaryotes probably possess mitochondria or organelles with a mitochondrial ancestry [1] . In fact, many eukaryotic lineages have mitochondria-derived organelles that deviate substantially from the textbook view of a mitochondrion as an oxygen-dependent organelle that produces large amounts of ATP [2] . The variations range from mitochondria-like organelles wherein alternative electron acceptors are used, to hydrogenosomes that use different energy-generating pathways and produce hydrogen under anaerobic conditions, and to mitosomes that have lost the energy-producing trait and the organellar genome [1] . Diplomonads are heterotrophic flagellates found in anaerobic/microaerobic habitats such as aquatic sediments or the digestive tract of animals. The human intestinal parasite Giardia intestinalis , the most-studied diplomonad, possesses mitosomes and show non-organellar subcellular localization of pyruvate ferredoxin oxidoreductase (PFOR) and [FeFe]-hydrogenase [3] , [4] , [5] . Other diplomonads of the genus Spironucleus have also been shown to encode [FeFe]-hydrogenase [6] and, recently, hydrogen production was reported to occur in the diplomonad Spironucleus vortens at a rate similar to the hydrogenosome-containing Trichomonas vaginalis and 40-fold higher than in G. intestinalis [7] . The basis of high-level hydrogen production and the evolutionary histories of the genetic components required have not been clarified. Here we describe the characterization of the mitochondria-related organelle (MRO) in Spironucleus salmonicida and provide evidence of a more complex organelle than the G. intestinalis mitosome using comparative genomics and proteomics of hydrogenosome-enriched fractions. We show that hydrogen production is prevalent in the genus Spironucleus during in vitro growth and display localization of the hydrogenase maturation machinery, PFOR and [FeFe]-hydrogenase to the MRO, evidence consistent with the organelle being a hydrogenosome. Phylogenetic reconstructions of hydrogenase maturases, [FeFe]-hydrogenases and PFORs support the presence of hydrogenosomes in the common ancestor of parabasalids and diplomonads. S. salmonicida harbours MROs We utilized our draft genome sequence of the salmon parasite S. salmonicida in combination with the recently developed stable transfection system for the parasite [8] to investigate the nature of its MROs and the origin, extent and basis for hydrogen production in Spironucleus . We constructed a S. salmonicida strain that carries a chromosomally integrated haemagglutinin (HA)-tagged Chaperonin 60 (Cpn60), a marker for MROs, and employed immunofluorescence to investigate its subcellular localization. Cpn60 localized to punctuate structures in the cytoplasm posterior to the nuclei ( Fig. 1a ). Transmission electron microscopy of these cells revealed electron-dense, double-membrane-bounded organelles characteristic of MROs ( Fig. 1b–d and Supplementary Fig. S1 ). The organelles are often round to ovoid and 300–400 × 200 nm in size, but variations in size and morphology are not uncommon ( Supplementary Figs S1 and S2 ). Immunoelectron microscopy using a HA epitope on Cpn60 and quantification of the gold labelling revealed 174 times higher labelling density of electron-dense organelles compared with the cell body (Supplementary Fig. S2s). The presence of double-membrane electron-dense organelles harbouring Cpn60 demonstrates the presence of MROs in S. salmonicida. 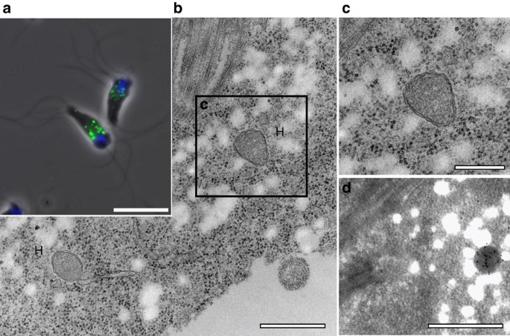Figure 1:Spironucleus salmonicidaharbours MROs. (a) A merged immunofluoresence and phase-contrast image ofS. salmonicidacells expressing Cpn60-3xHA. The epitope-tagged protein is detected by monoclonal anti-HA Alexa Fluor 488 (green). Nuclei are labelled with DAPI (4',6-diamidino-2-phenylindole, blue). Scale bar, 10 μm. (b) Two double-membraned organelles (H) in a transmission electron micrograph of anS. salmonicidacell expressing Cpn60-3xHA. Scale bar, 500 nm. (c) Enlarged view of the double-membraned organelle marked by a black box inb. Scale bar, 250 nm. (d) Immunoelectron microscopy performed towards the HA epitope inS. salmonicidacells expressing Cpn60-3xHA decorates electron-dense organelles with gold label, consistent with the organelle harbouring Cpn60 and being an MRO (scale bar, 500 nm). Figure 1: Spironucleus salmonicida harbours MROs. ( a ) A merged immunofluoresence and phase-contrast image of S. salmonicida cells expressing Cpn60-3xHA. The epitope-tagged protein is detected by monoclonal anti-HA Alexa Fluor 488 (green). Nuclei are labelled with DAPI (4',6-diamidino-2-phenylindole, blue). Scale bar, 10 μm. ( b ) Two double-membraned organelles (H) in a transmission electron micrograph of an S. salmonicida cell expressing Cpn60-3xHA. Scale bar, 500 nm. ( c ) Enlarged view of the double-membraned organelle marked by a black box in b . Scale bar, 250 nm. ( d ) Immunoelectron microscopy performed towards the HA epitope in S. salmonicida cells expressing Cpn60-3xHA decorates electron-dense organelles with gold label, consistent with the organelle harbouring Cpn60 and being an MRO (scale bar, 500 nm). Full size image We searched the draft genome sequence of S. salmonicida for proteins involved in mitochondrion-derived machineries, such as oxidative phosphorylation, Fe–S cluster biogenesis [9] and organelle protein translocation in MROs. We were unable to detect any proteins involved in oxidative phosphorylation, indicating that the MRO of S. salmonicida is not a mitochondrial-like organelle similar to those in Blastocystis [10] . Several homologues of genes predicted to be involved in MRO Fe–S cluster biosynthesis (IscU, IscS, Nfu, frataxin and two ferredoxins), protein import and homeostasis (Tom40, Pam18, HSP70, Jac1 and GrpE) were identified in the S. salmonicida genome and were shown to localize with Cpn60 to the MROs ( Supplementary Fig. S3 and Supplementary Table S1 ). All the above genes, except frataxin, are present in the G. intestinalis genome and the proteins are known to localize to the mitosome [11] , [12] , [13] , [14] . We failed to detect homologues of the α- or β-subunits of the mitochondrial processing peptidase in the S. salmonicida genome and, accordingly, none of the proteins that localized to the MRO carried putative amino-terminal targeting peptides ( Supplementary Fig. S4 ). Despite this absence, the Giardia mitosomal import machinery was able to recognize and import an HA-tagged S. salmonicida Pam18 when expressed in G. intestinalis ( Supplementary Fig. S5 ). Hydrogen production is prevalent in Spironucleus We investigated whether hydrogen production is restricted to S. vortens or whether other Spironucleus species also can evolve hydrogen. S. salmonicida , S. barkhanus and S. vortens were grown at their preferred growth temperatures for 48 h in air-tight glass vials before samples of the gaseous phase were analysed by gas chromatography. All three Spironucleus species were found to produce molecular hydrogen at high levels, with S. vortens producing the highest amounts ( Fig. 2a ), eight- to tenfold higher than S. salmonicida and S. barkhanus ( Fig. 2a ). Hydrogen production in G. intestinalis , although measured previously by membrane inlet mass spectrometry [4] , was below the detection level of the method employed in this work. 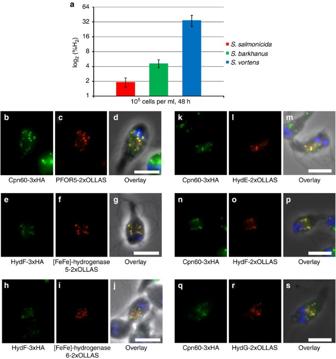Figure 2: Hydrogen production inSpironucleusand evidence of hydrogenosomes inSpironucleus salmonicida. (a) Hydrogen production was assayed in three strains ofSpironucleus(S. salmonicida,S. barkhanusandS. vortens). The percentage of hydrogen gas in the head-space of cultures (%H2) after 48 h of growth from 105cells per ml at the prefered growth temperature (S. salmonicida16 °C,S. barkhanus4 °C andS. vortens22 °C) was recorded. The log2(%H2) is plotted for each strain. All three strains produce hydrogen, withS. vortensproducing eight- to tenfold higher amounts thanS. salmonicidaandS. barkhanus. Error bars indicate s.d. (n=3). AnS. salmonicidacell expressing (b) Cpn60-3xHA (green) and (c) PFOR5-2xOLLAS (red). (d) Merged imaged ofbandc, with DAPI (4',6-diamidino-2-phenylindole)-labelled nuclei (blue) and phase-contrast image show colocalization of the green and red label. AnS. salmonicidacell expressing (e) HydF-3xHA (green) and (f) [FeFe]-hydrogenase 5-2xOLLAS (red). (g) Merged imaged ofeandfshow colocalization of the green and red label. AnS. salmonicidacell expressing (h) HydF-3xHA (green) and (i) [FeFe]-hydrogenase 6-2xOLLAS (red). (j) Merged imaged ofhandidisplay colocalization of the green and red label. AnS. salmonicidacell expressing (k) Cpn60-3xHA (green) and (l) HydE-2xOLLAS (red). (m) Merged imaged ofkandldemonstrate colocalization of the green and red label. AnS. salmonicidacell expressing (n) Cpn60-3xHA (green) and (o) HydF-2xOLLAS (red). (p) Merged imaged ofnandoshow colocalization of the green and red label. AnS. salmonicidacell expressing (q) Cpn60-3xHA (green) and (r) HydG-2xOLLAS (red). (s) Merged imaged ofqandrshow colocalization of the green and red label. (all scale bars 5 μm). Figure 2: Hydrogen production in Spironucleus and evidence of hydrogenosomes in Spironucleus salmonicida. ( a ) Hydrogen production was assayed in three strains of Spironucleus ( S. salmonicida , S. barkhanus and S. vortens ). The percentage of hydrogen gas in the head-space of cultures (%H 2 ) after 48 h of growth from 10 5 cells per ml at the prefered growth temperature ( S. salmonicida 16 °C, S. barkhanus 4 °C and S. vortens 22 °C) was recorded. The log 2 (%H 2 ) is plotted for each strain. All three strains produce hydrogen, with S. vortens producing eight- to tenfold higher amounts than S. salmonicida and S. barkhanus . Error bars indicate s.d. ( n =3). An S. salmonicida cell expressing ( b ) Cpn60-3xHA (green) and ( c ) PFOR5-2xOLLAS (red). ( d ) Merged imaged of b and c , with DAPI (4',6-diamidino-2-phenylindole)-labelled nuclei (blue) and phase-contrast image show colocalization of the green and red label. An S. salmonicida cell expressing ( e ) HydF-3xHA (green) and ( f ) [FeFe]-hydrogenase 5-2xOLLAS (red). ( g ) Merged imaged of e and f show colocalization of the green and red label. An S. salmonicida cell expressing ( h ) HydF-3xHA (green) and ( i ) [FeFe]-hydrogenase 6-2xOLLAS (red). ( j ) Merged imaged of h and i display colocalization of the green and red label. An S. salmonicida cell expressing ( k ) Cpn60-3xHA (green) and ( l ) HydE-2xOLLAS (red). ( m ) Merged imaged of k and l demonstrate colocalization of the green and red label. An S. salmonicida cell expressing ( n ) Cpn60-3xHA (green) and ( o ) HydF-2xOLLAS (red). ( p ) Merged imaged of n and o show colocalization of the green and red label. An S. salmonicida cell expressing ( q ) Cpn60-3xHA (green) and ( r ) HydG-2xOLLAS (red). ( s ) Merged imaged of q and r show colocalization of the green and red label. (all scale bars 5 μm). Full size image Hydrogenosomes are present in S. salmonicida The molecular basis for hydrogen production in S. salmonicida was investigated by bioinformatic searches in the draft genome sequence that revealed a set of five PFORs and seven [FeFe]-hydrogenases. Out of the five PFORs, only PFOR5 displayed MRO localization by epitope tagging and immunostaining ( Fig. 2b–d ), whereas the remaining four PFORs displayed either localization to the cytoplasm or a potential membrane association. Studying the subcellular localizations of epitope-tagged [FeFe]-hydrogenases revealed that FeHyd5 and FeHyd6 displayed MRO localization ( Fig. 2e–j ). The other hydrogenases were found to have diffuse localization to the cytoplasm. The presence of homologues of PFOR and [FeFe]-hydrogenase in the MRO and the cytoplasm suggests cytoplasmic and organellar hydrogen production. In other species, the active site of [FeFe]-hydrogenase carries an organometallic H-cluster, and maturation of the 2Fe subcluster is believed to be carried out by the hydrogenase maturases HydEFG [15] , [16] . We identified single-copy homologues of HydE, HydF and HydG in the genome of S. salmonicida . The localizations of the three maturases were investigated by epitope tagging and they colocalized with Cpn60 in the MRO of S. salmonicida ( Fig. 2k–s ). Direct interactions of HydG–HydF and HydF–HydF were observed by an in situ proximity ligation assay (PLA) using antibodies against the HA and OLLAS epitope tags ( Supplementary Fig. S6 ). PLA also provided evidence for interaction of the scaffold protein HydF with FeHyd2, FeHyd5 and FeHyd6. We have not been able to colocalize FeHyd2 with HydF to hydrogenosomes to confirm the authenticity of this interaction, but the interactions of FeHyd5 and FeHyd6 with HydF are in agreement with their mutual localization to the MRO ( Supplementary Fig. S6 ). Evolutionary origin of hydrogenosomes in S. salmonicida We assembled amino acid sequence data sets of PFOR, [FeFe]-hydrogenase and the hydrogenase maturases, which included homologues from S. salmonicida , S. vortens and the free-living diplomonad Trepomonas sp. PC1, and performed maximum likelihood (ML) and Bayesian inference phylogenetic analyses ( Fig. 3 and Supplementary Figs S7–S11 ). The diplomonads are monophyletic in all three hydrogenase maturase trees ( Fig. 3 ), suggesting that they were present in their common ancestor. HydF ( Fig. 3b ) and HydG ( Fig. 3c ) show monophyletic eukaryotes, whereas the diplomonad HydE ( Fig. 3a .) sequences branch weakly with two bacterial homologues as a sister group to the rest of the eukaryotes in the ML tree. However, monophyly of the eukaryotes is also supported for the HydE data set in the Bayesian analysis. The topologies of the three trees are consistent with the presence of hydrogenase maturases in the common ancestor of diplomonads and parabasalids. 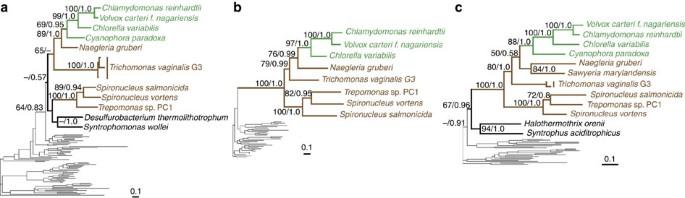Figure 3: Phylogenies of hydrogenase maturases HydEFG. Phylogenies of (a) HydE, (b) HydF and (c) HydG inferred from ML analyses.S. salmonicidahomologues that localize to the hydrogenosome are indicated by bold font. ML bootstrap values and Bayesian inference posterior probabilities are shown for bipartitions with support greater than 50% and 0.5, respectively. Excavata and Plantae sequences are coloured brown and green, respectively. Black branches indicate prokaryotic sequences. SeeSupplementary Figs S9-S11, S13 and S15for detailed phylogenies. Figure 3: Phylogenies of hydrogenase maturases HydEFG. Phylogenies of ( a ) HydE, ( b ) HydF and ( c ) HydG inferred from ML analyses. S. salmonicida homologues that localize to the hydrogenosome are indicated by bold font. ML bootstrap values and Bayesian inference posterior probabilities are shown for bipartitions with support greater than 50% and 0.5, respectively. Excavata and Plantae sequences are coloured brown and green, respectively. Black branches indicate prokaryotic sequences. See Supplementary Figs S9-S11, S13 and S15 for detailed phylogenies. Full size image The PFOR phylogeny also shows monophyletic eukaryotes, where the diplomonad sequences are found in two clusters within a group containing the T. vaginalis sequences ( Supplementary Fig. S7 ). The topology within this group is consistent with the presence of four paralogues in the common ancestor of diplomonads. Two of the paralogues (III and IV) have been lost in the lineage leading to Giardia , including the orthologue of PFOR5 that shows localization to the S. salmonicida hydrogenosome ( Supplementary Fig. S7 ). The phylogeny of [FeFe]-hydrogenase is more complex and difficult to interpret. Nevertheless, it suggests the presence of multiple paralogues in the diplomonad ancestor, rather than a recent lineage-specific expansion ( Supplementary Fig. S11 ). The parabasalid hydrogenases are found in two groups in a different part of the tree with weak support, indicating that a common ancestry is plausible. Taken together, the phylogenies support a common origin of the key components of the hydrogenosome in parabasalids and diplomonads. The S. salmonicida hydrogenosomes contain metabolic genes The S. salmonicida genome sequence was found to contain homologues of many T. vaginalis hydrogenosomal proteins [17] . The subcellular localizations of 20 of these proteins were investigated by epitope tagging ( Supplementary Tables S2 and S3 ) and revealed two more proteins that localized to the S. salmonicida hydrogenosome: a potential H-protein of the glycine decarboxylase complex ( Supplementary Fig. S12a-c ) and serine hydroxylmethyltransferase (SHMT, Supplementary Fig. S12d–f ). Both proteins lack orthologous genes in the G. intestinalis genomes but are localized to the hydrogenosomes of T. vaginalis [18] , [19] . The diplomonad homologues of SHMT are monophyletic and branch earliest within the eukaryotic cluster with Trichomonas as the next branch ( Supplementary Fig. S13 ). This is consistent with a non-recent origin of this hydrogenosome-targeted enzyme in S. salmonicida. The presence of SHMT and a potential H-protein of the glycine decarboxylase complex argues for amino acid metabolism in the hydrogenosome of S. salmonicida . Insight into hydrogenosome function by proteomics We adapted a cellular fractionation protocol developed to enrich for Giardia mitosomes [3] and applied it to S. salmonicida to enrich for hydrogenosomes, and thereby identify and expand the list of hydrogenosome-targeted proteins. Subcellular fractions of Cpn60-3xHA-expressing cells were established by differential centrifugation and a discontinuous Nycodenz gradient, followed by the identification of hydrogenosome-enriched fractions by western blotting ( Fig. 4a,b ). We subjected two Nycodenz gradient fractions, N1 and N3, the latter enriched in hydrogenosomes, as well as the starting material to the Nycodenz gradient (P50) to proteomic analysis by liquid chromatography tandem mass spectrometry (LC–MS/MS) and matched the peptides against the S. salmonicida proteome using Mascot [20] . In total, 2,973 peptides matching 803 proteins were detected in the hydrogenosome-enriched fraction, including the majority of proteins in the different proposed hydrogenosomal pathways ( Supplementary Table S1 and Supplementary Data 1 ). In an effort to identify novel hydrogenosomal proteins, we used the presence or absence of proteins in the three different fractions to establish candidates for colocalization experiments ( Fig. 4c ). Nine of the verified hydrogenosomal proteins are exclusively detected in the N3 fraction, five hydrogenosomal proteins are found in N3 and P50, and three are detected across all three fractions ( Fig. 4c ). On the basis of these observations, we picked seven candidates exclusively detected in the hydrogenosome-enriched fraction, four candidates found in N3 and P50, and the last candidate was found across all three fractions. The subcellular localizations of these proteins were established by immunofluorescence experiments ( Supplementary Fig. S14 ). Five of the candidate proteins, derived from all three categories, were found to display a subcellular localization consistent with endoplasmic reticulum in S. salmonicida [8] . One of the chosen proteins of the hydrogenosome-enriched fraction, a divergent paralogue of acetyl-CoA synthetase (ADP-forming), was found to display a hydrogenosomal localization ( Fig. 4d–g ). Phylogenetic analysis of the hydrogenosomal acetyl-CoA synthetase shows polyphyletic eukaryotes, probably because of repeated gene transfer events ( Supplementary Fig. S15 ), as previously suggested [21] . Interestingly, the presence of an acetyl-CoA synthetase in the hydrogenosome could complete a minimal hypothetical pathway from pyruvate to acetate ( Fig. 5 ). We hypothesize that electrons are removed from pyruvate by PFOR5 and then shuttled by one or both of the organellar ferredoxins to the hydrogenases, which reoxidize the ferredoxin with the concomitant production of molecular hydrogen. Pyruvate is converted into acetyl-CoA and CO 2 by PFOR and the former is used by acetyl-CoA synthetase (ADP-forming) to generate ATP from ADP. The end products from this metabolic scheme will be CO 2 , acetate and H 2 ( Fig. 5 ). Unfortunately, no experimental data describing the metabolism is available for S. salmonicida , but the proposed end products were identified as the major end products of S. vortens metabolism [22] . 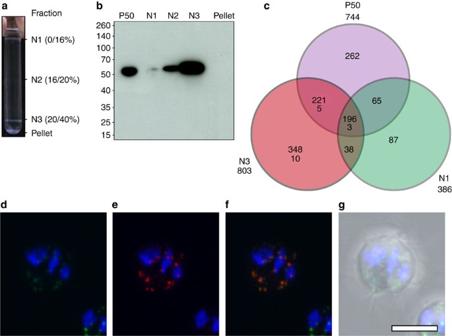Figure 4: Proteomic analyses of a hydrogenosome-enriched fraction. (a) Nycodenz discontinuous gradient for the preparation of a hydrogenosome-enriched fraction starting from fraction P50. The Nycodenz interfaces are indicated along with the corresponding fraction or pellet designation. (b) Western Blot of recovered fractions fromain addition to the P50 fraction, which is the starting material for the Nycodenz discontinuous gradient. Hydrogenosomes are detected in P50 and in fractions N2 and N3, with N3 containing the largest amount of epitope-tagged Cpn60. (c) Venn-diagram showing common and differential distribution of proteins identified by LC–MS/MS in fractions P50, N1 and N3. The total number of proteins identified in each fraction is displayed below the fraction designation in bold. The distribution of verified hydrogenosomal proteins in the fractions is indicated below the total number of identified proteins if applicable. (d) AS. salmonicidacell expressing 3xHA-tagged HydF (green). Nuclei are labelled with DAPI (4',6-diamidino-2-phenylindole, blue). (e) Same cell as ind, stained for 2xOLLAS-tagged acetyl-CoA synthetase. (f) Merged image ofdande. (g) DIC image merged withd–f. HydF and acetyl-CoA synthetase colocalize to the hydrogenosome. The cell was imaged by laser-scanning confocal microscopy. Scale bar, 5 μm. Figure 4: Proteomic analyses of a hydrogenosome-enriched fraction. ( a ) Nycodenz discontinuous gradient for the preparation of a hydrogenosome-enriched fraction starting from fraction P50. The Nycodenz interfaces are indicated along with the corresponding fraction or pellet designation. ( b ) Western Blot of recovered fractions from a in addition to the P50 fraction, which is the starting material for the Nycodenz discontinuous gradient. Hydrogenosomes are detected in P50 and in fractions N2 and N3, with N3 containing the largest amount of epitope-tagged Cpn60. ( c ) Venn-diagram showing common and differential distribution of proteins identified by LC–MS/MS in fractions P50, N1 and N3. The total number of proteins identified in each fraction is displayed below the fraction designation in bold. The distribution of verified hydrogenosomal proteins in the fractions is indicated below the total number of identified proteins if applicable. ( d ) A S. salmonicida cell expressing 3xHA-tagged HydF (green). Nuclei are labelled with DAPI (4',6-diamidino-2-phenylindole, blue). ( e ) Same cell as in d , stained for 2xOLLAS-tagged acetyl-CoA synthetase. ( f ) Merged image of d and e . ( g ) DIC image merged with d – f . HydF and acetyl-CoA synthetase colocalize to the hydrogenosome. The cell was imaged by laser-scanning confocal microscopy. Scale bar, 5 μm. 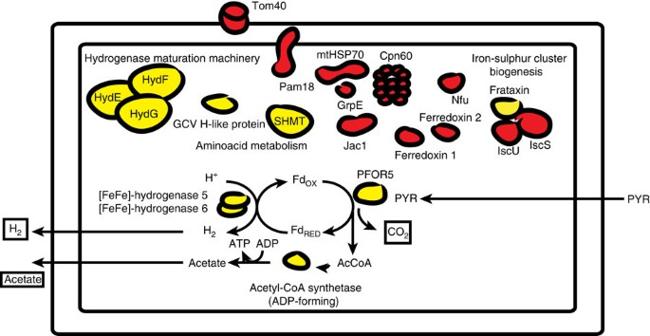Figure 5: The minimal hydrogenosomal proteome inS. salmonicidaindicate a hypothetical organellar pyruvate metabolism. Proteins identified in both the mitosome ofG. intestinalisand the hydrogenosome ofS. salmonicidaare shown in red. Proteins identified in theS. salmonicidahydrogenosome but not in theG. intestinalismitosome are shown in yellow. Potential end products of hydrogenosome metabolism are in boxes. FdOX, FdRED, oxidized and reduced ferredoxin; AcCoA, acetyl-CoA, PFOR, pyruvate ferredoxin oxidoreductase; SHMT, serine hydroxylmethyltransferase; GDC, glycine decarboxylase complex; PYR, pyruvate. Full size image Figure 5: The minimal hydrogenosomal proteome in S. salmonicida indicate a hypothetical organellar pyruvate metabolism. Proteins identified in both the mitosome of G. intestinalis and the hydrogenosome of S. salmonicida are shown in red. Proteins identified in the S. salmonicida hydrogenosome but not in the G. intestinalis mitosome are shown in yellow. Potential end products of hydrogenosome metabolism are in boxes. Fd OX , Fd RED , oxidized and reduced ferredoxin; AcCoA, acetyl-CoA, PFOR, pyruvate ferredoxin oxidoreductase; SHMT, serine hydroxylmethyltransferase; GDC, glycine decarboxylase complex; PYR, pyruvate. Full size image Several observations argue for the presence of hydrogen-producing organelles in the diplomonad ancestor. First, we confirm the presence of hydrogen production in S. vortens [7] and showed that also S. salmonicida and S. barkhanus produces hydrogen at a higher rate than G. intestinalis ( Fig. 2a ). Second, two key components of hydrogenosomes, [FeFe]-hydrogenase and PFOR, were shown to be present in the S. salmonicida organelle ( Fig. 2b–d ). The phylogenetic reconstructions showed that these hydrogenosome-targeted proteins represent diplomonad paralogues present in the free-living diplomonad Trepomonas sp. PC1, but not the hydrogenosome-lacking human parasite G. intestinalis ( Fig. 3 and Supplementary Figs S7 and S11 ). Third, the hydrogenase maturation machinery was shown to localize to the hydrogenosome in S. salmonicida similar to that in T. vaginalis [23] ( Fig. 2k–s ). Phylogenies of the three maturase proteins indicate early origins that predate the split of Fornicata and Parabasalia ( Fig. 3 ). Fourth, homologues of two hydrogenosomal proteins involved in amino acid metabolism in T. vaginalis were shown to be present in the S. salmonicida hydrogenosome ( Supplementary Fig. S12 ). Finally, relatives of diplomonads within Fornicata exhibit double-membrane organelles reminiscent of the hydrogenosomes of Spironucleus and parabasalids [24] , [25] . These results point to that the common ancestor of Fornicata and parabasalids harboured hydrogenosomes, and it suggests that G. intestinalis mitosomes have evolved from hydrogenosomes. Functional and evolutionary studies of additional MROs of metamonads and other microbial eukaryotes are needed to evaluate the evolutionary role of metamonads in the establishment of hydrogen metabolism in eukaryotes and to reveal the full spectrum of MROs. Reagents and cell culture Unless otherwise indicated, the reagents were obtained from Sigma Chemical Co., USA. S. salmonicida (ATCC 50377, previously ATCC 50380), S. barkhanus [26] and S. vortens (ATCC 50386) were obtained from the American Type Culture Collection (ATCC) and grown in axenic cultures in modified LYI culture media [8] at 16, 4 and 22 °C, respectively. G. intestinalis isolate WB clone C6 (ATCC 50803) was cultivated in TYDK media at 37 °C in 10 ml tightly capped slanted culture tubes (NUNC) [27] . Generation and maintenance of transfectants Transfection and maintenance of S. salmonicida transfectants followed the methods described in Jerlström-Hultqvist et al . [8] Briefly, one confluent tube of S. salmonicida cells (~10 6 cells per ml) was placed in ice slush 15 min and repeatedly tapped to detach the cells. The cells were pelleted by centrifugation (500 g , 5 min, 4 °C) and the supernatant was aspirated. The cells were resuspended to a concentration of ~10 7 cells per ml in ice-cold LYI media and 300 μl of the cell suspension was distributed in a 0.4-cm gap cuvette (Bio-Rad). Circular (20–50 μg) or linearized plasmid DNA (15–20 μg) in a volume not larger than 30 μl was added to the cells and electroporation was performed using a GenePulser (Bio-Rad) with a capacitance extender set at 320 V, 800 Ω and 960 μF. Post transfection, the cuvettes were moved to ice slush 10–15 min before being transferred to fresh temperated LYI media containing 50 μg ml −1 gentamicin (Gibco). The cells were incubated at 16 °C for 24 h before selection was applied (puromycin, 50 μg ml −1 ; blasticidin S, 20 μg ml −1 and G418, 150 μg ml −1 ). Fresh media and selective drug was replaced weekly until confluence. Transfectants were maintained under continuous selection and passaged weekly. Double-transfectants were generated as described above for the wild-type, but employing a transfected recipient strain instead. Transfectants involving simultaneous puromycin and blasticidin S selection necessitated the use of 80 μg ml −1 of the latter drug for efficient selection. Transfection of G. intestinalis was performed as described for S. salmonicida , except that TYDK growth media was used, the electroporator was set at 350 V, 800 Ω and 960 μF, and cells were maintained at 37 °C. G. intestinalis transfectants were selected and maintained using 50 μg ml −1 puromycin [28] . Transmission electron microscopy S. salmonicida cells carrying an integrated Cpn60-3xHA construct were fixed in 2% glutaraldehyde and 1% paraformaldehyde in 0.1 M cacodylate buffer, pH 7.4, and stored in refrigerator. After fixation, cells were rinsed in 0.1 M phosphate buffer and centrifuged. The pellets were then postfixed in 2% osmium tetroxide in 0.1 M phosphate buffer, pH 7.4, at 4 °C for 2 h, dehydrated in ethanol followed by acetone and embedded in LX-112 (Ladd, Burlington, VT, USA). Ultrathin sections (~40–50 nm) were cut by a Leica EM UC 6 (Leica, Wien, Austria). Sections were contrasted with uranyl acetate followed by lead citrate and examined in a Tecnai 12 Spirit Bio TWIN transmission electron microscope (FEI Company, Eindhoven, The Netherlands) at 100 kV. Digital images were taken by using a Veleta camera (Olympus Soft Imaging Solutions, GmbH, Münster, Germany). Immunoelectron microscopy S. salmonicida transfectants carrying an integrated Cpn60-3xHA construct were fixed in 2% glutaraldehyde (G5882, Sigma-Aldrich) and 1% paraformaldehyde (00380, Polysciences) in 0.1 M sodium cacodylate, pH 7.4, at 4 °C for at least 24 h for EPON embedding. Cells for Lowicryl embedding were fixed in 4% paraformaldehyde and 0.2% glutaraldehyde in 0.1 M sodium cacodylate, pH 7.4, at 4 °C for at least 24 h. Cells for EPON embedding were incubated in 0.1% osmium tetroxide for 1 min and then washed with 0.1 M cacodylate, pH 7.4. The cells were dehydrated in 70% EtOH for 30 min, followed by 95% for 30 min and finally in absolute ethanol for 2 × 15 min. The cell pellet was incubated with EPON resin with agar for 30 min. The plastic was exchanged and the sample incubated 4 h at room temperature. New EPON resin was added and the samples were incubated overnight at room temperature. The samples were polymerized at 60 °C for 2 days and ultrathin slices of 50-60 nm were prepared in an ultramicrotome (LKB ultratome V). The slices were etched in metaperiodate 10 min at room temperature followed by 3 × 5 min washes in H 2 O. For Lowicryl embedding, the cells were dehydrated as described above and incubated 1 h each of a 1:2 and then 1:1 mixture of Lowicryl K4M and absolute ethanol followed by Lowicryl only for 1 h. The plastic was exchanged and incubated 2 h followed by a fresh exchange of resin for 16 h. The plastic was ultraviolet-polymerized at −20 °C for 2 days followed by 1 day in ambient light. Slices were prepared as for the EPON resin. The slices were blocked in 3% BSA for 30 min at room temperature followed by overnight incubation at 4 °C with the anti-HA monoclonal antibody (H9658, Sigma-Aldrich; 1:200). The slices were washed in Tris-buffered saline for 3 × 5 min and incubated with the anti-mouse 10 nm colloidal gold antibody (Biosensis) for 2 h at room temperature. The slices were washed as described above and contrasted using 5% uranyl acetate for 20 min and lead nitrate for 2 min according to Reynolds [29] . The slices were dried and mounted for electron microscopy before being viewed in a Hitachi H-7100 electron microscope operating at 75 kV. ImageJ [30] was used to calculate gold labelling densities in cellular compartments from electron micrographs of immunogold labelled Lowicryl sections. Measurement of H 2 production The cell cultures were placed in ice slush for 15 min and the cell densities counted in a haemocytometer. The cultures were pelleted (500 g , 5 min, 4 °C) and resuspended in their respective preferred growth media to a density of 10 5 or 10 6 cells per ml. Glass tubes (125 × 10-SV T047, Chromacol) with screw-caps (500 × 12-SC, Chromacol) and insert membranes (500 × 12-6RT1, Chromacol) for sampling of the gaseous phase were inoculated in triplicates using 6 ml of the cell suspensions. The tubes were incubated at the preferred growth temperature ( S. salmonicida 16 °C, S. barkhanus 4 °C, S. vortens 22 °C and G. intestinalis 37 °C) for 24 or 48 h. The gaseous phase was sampled by withdrawing 100 μl of gas with a Hamilton syringe and then injected into a Clarus 500 (Perkin Elmer) bench-top GC equipped with a molecular sieve 5 A 60/80 mesh column (Perkin Elmer) employing argon as the carrier gas. The integrated peak areas were used to calculate the H 2 content of the gas. A standard curve was constructed by measuring known volumetric H 2 ratios and this was used to estimate the hydrogen gas in the measured samples. Immunofluorescence Cells in culture tubes were placed in ice slush 15 min to detach cells, moved to 15 ml Falcon tubes and pelleted by centrifugation (500 g , 5 min, 4 °C). The supernatant was aspirated and the cells were washed with at least ten pellet volumes of ice-cold HEPES-buffered saline with added glucose [8] before being applied to polylysine-coated slides (Thermo Scientific, ER-208B-AD-CE24). The cells were fixed in 2% paraformaldehyde in PBS for 20 min at 37 °C. Two washes with PBS were performed and the cells were then quenched for 10 min using 0.1 M glycine in PBS at room temperature. The quenching solution was removed, the cells were washed twice with PBS and permeabilized for 30 min at room temperature using 0.2% Triton X-100 in PBS. The cells were blocked in antibody block solution (2% BSA in PBS) either overnight at 4 °C or 1 h at room temperature. The proteins with 3xHA or 2xOLLAS tags were detected by an anti-HA monoclonal mouse antibody (H9658, Sigma-Aldrich, 1:1,000) or an OLLAS tag Antibody (A01658, GenScript, 1:2,000), respectively. The primary antibodies were detected by polyclonal goat anti-mouse Alexa Fluor 488 (A-11001, Life Technologies, 1:250) or goat anti-rabbit Alexa Fluor 594 (A-11037, Life Technologies, 1:250), respectively. Alternatively, the 3xHA tag was detected by HA.11 Clone 16B12 Monoclonal Antibody, Alexa Fluor 488 Labeled (A488-101 L, Covance, 1:250). All antibodies were diluted in antibody block solution. The cells were mounted in Vectashield containing DAPI (H-1200, Vector Labs) and examined with a Zeiss Axioplan2 fluorescence microscope or a Zeiss 510 laser-scanning confocal microscope. Images were processed using the software AxioVision LE Rel. 4.8.2.0 or Zen 2011 v7.0.0.285 (Carl Zeiss GmbH). Cloning of genes into tagging vectors The coding sequences and an additional 200–500 bp upstream sequence were PCR amplified from genomic DNA of S. salmonicida ( Supplementary Table S1 ) using Phusion Hot Start II High-fidelity DNA polymerase (Phusion HS II) (Thermo Scientific). Oligonucleotides targeting the genes were designed according to the Phusion HS II manufacturer’s recommendations and introduced unique terminal restriction sites for cloning ( Supplementary Table S2 ) into the multiple cloning site of the pSpiro suite of vectors with a carboxy-terminal epitope tag [8] . The amplified gene fragments were purified, digested using standard methods and cloned into the appropriate pSpiro vector [8] ( Supplementary Table S3 ). The S. salmonicida Pam18 for expression in G. intestinalis was resynthesized using a modified Simplified Gene Synthesis protocol employing Phusion HS II and the constructed gene was introduced into the G. intestinalis AC expression vector [28] . The sequence of the constructed vectors was verified by Sanger sequencing. Identification of candidate MRO sequences in S. salmonicida Verified mitosomal proteins from G. intestinalis and verified hydrogenosomal proteins [5] , [12] , [13] , [14] , [17] , [18] , [19] , [31] , [32] from T. vaginalis were downloaded from GiardiaDB [33] and TrichDB [33] , respectively, and were used to query draft-proteomes or -genome sequences of S. salmonicida by reciprocal BLASTP and TBLASTN searches. Phylogenetic analyses Dataset representing the sampled diversity of PFOR, hydrogenase maturases, [FeFe]-hydrogenase, SHMT and acetyl CoA synthetase (ACS) were assembled. The S. vortens database [34] and our transcriptome data on Trepomonas sp. PC1 were mined and identified homologous proteins were added. The data sets were aligned using MUSCLE, version 3.8.31 (ref. 35 ). Unambiguously aligned regions were manually identified. ML trees were generated using RAxML, version 7.3.0 (ref. 36 ). An algorithm that searches for the best-scoring ML tree and performs a rapid bootstrap analysis with 1,000 bootstrap replicates in one single run was applied (-f a -# 1000). The PROTCATWAG model for amino acid substitution was used in all ML analyses. MrBayes, version 3.2.1 (ref. 37 ), was used on the same alignments and the mixed amino acid substitution model with γ-rates to generate Bayesian inference posterior probabilities. Two simultaneous analyses each with four chains were run for 4,000,000 (PFOR) or 2,000,000 (all other data sets) generations, with a relative burnin fraction of 25%. See Supplementary Figs S7–S11, S13 and S15 for further details. In situ PLA assay Cells for in situ PLA assays were prepared and fixed as described in the immunofluorescence section. Cells were blocked overnight in 1xDuoLink Block solution and co-incubated with anti-HA mouse monoclonal (H9658, Sigma-Aldrich; 1:1,000) and rabbit polyclonal OLLAS tag Antibody (A01658, GenScript; 1:2,000) in antibody diluent (Olink Biosciences) for 2 h at room temperature in a humidified chamber. The primary antibodies were omitted either individually or altogether in some reactions to monitor the amounts of background amplification. PLA probe decoration, proximity ligation and rolling-circle amplification followed the instruction in the DuoLink In Situ user manual (Olink Biosciences). The slides were viewed using a Zeiss Axioplan2 fluorescence microscope or a Zeiss 510 laser-scanning confocal microscope. Images were analysed using BlobFinder v3.2 (ref. 38 ) to extract the number of PLA signals and cell nuclei. At least 500 cells were counted for any given experiment and cell line. SigmaPlot12 (Systat Software) was used to investigate normal distribution (Shapiro–Wilks test) and equal variance of the PLA signal to the number of nuclei. Multiple comparison analysis of variance with Holm–Sidăk test (α-level 0.05) as implemented in SigmaPlot12 was used to determine statistical significance from three biological replicates. Partial purification of S. salmonicida hydrogenosomes S. salmonicida cells expressing Cpn60-3xHA used for purification were grown in 1,000 ml LYI medium divided into 50 ml falcon tubes at 16 °C for 5–7 days. The following protocol of purification is an adaption from Emelyanov et al . [3] All the following steps were performed at 4 °C, unless otherwise stated. The cells were pelleted at 500 g for 5 min and the pellets were pooled and washed twice (500 g for 5 min) with 30 ml of isoHSDP (10 mM Hepes–KOH, 0.25 M sucrose pH 7.2) containing proteinase inhibitors to a final concentration of leupeptin 0.01 mg ml −1 , TLCK ( N -tosyl-l-lysine chloromethyl ketone) 0.05 mg ml −1 , phenylmethyl sulphonyl fluoride 0.1 mM and dithiothreitol (DTT) 4 mM. The cell pellet was dissolved in 6 ml of isoHSDP with protease inhibitors and the cells were counted in a Bürker chamber (2-3 × 10 8 cells per ml). The cell suspension was transferred to aliquots of 500 μl, snap-frozen in liquid N 2 and kept at −80 °C. Two to four millilitres of cell suspension from −80 °C were thawed on ice and 5 ml isoHSDP buffer with 4 mM DTT and 2 × protease inhibitors (complete, EDTA-free protease inhibitor cocktail, Roche) were added for each millilitre of cell suspension. To lyse the cells, sonication for 2 × 15 s on an ice bath was applied. To validate the extent of breakage, the cell suspension was monitored under light microscope. To remove nuclei and cell debris, the cell suspension was first centrifuged at 3,000 g for 20 min with an additional centrifugation of the supernatant at 5,600 g for 30 min. The supernatant was centrifuged at 50,000 g for 1 h 10 min (Sorvall, rotor S80-AT3) and the resulting pellet was resuspended in 6 ml isoHSDP with 4 mM DTT and protease inhibitors (complete, EDTA-free protease inhibitor cocktail) and re-pelleted at 50,000 g for 1 h 10 min. The resulting pellet (sample P50) was resuspended in 1 ml isoHSDP and layered on top off a discontinuous 16, 20 and 40% (w/v) Nycodenz (Axis-Shield) gradient, prepared with isoHSDP, 4 mM DTT and protease inhibitors (complete, EDTA-free protease inhibitor cocktail), and centrifuged (Kontron, rotor TST 41.14) at 36,000 g for 2 h 10 min. The three visible bands denoted N1, N2 and N3 (from the top to the bottom of the tube) were collected and diluted seven times with isoHSDP, and pelleted at 100,000 g for 40 min. The pellets were resuspended in 200 μl isoHSDP with 4 mM DTT and protease inhibitors (complete, EDTA-free protease inhibitor cocktail), quickly frozen in liquid nitrogen and stored at −80 °C. The three fractions (N1, N2 and N3) were analysed by western blotting using antibodies against the 3xHA-tagged hydrogenosomal marker Cpn60. Western blot Protein samples were separated by Tris-glycine SDS–PAGE using 5% stacking and 10% resolving gels and transferred by semidry blotting to BioTrace PVDF membranes (Pall Corporation) [28] . Polyvinylidene difluoride membranes were blocked in either 1% BSA in PBS–0.1% Tween 20 for detection of HA tag or 5% milk in PBS–0.1% Tween 20 for the OLLAS tag. The 3xHA- or 2xOLLAS-tagged proteins were detected by anti-HA monoclonal mouse antibody (H9658, Sigma-Aldrich, 1:10,000) or OLLAS Epitope Tag Antibody (NBP1-06713, Novus Biologicals, 1:1,000), respectively. The anti-HA and anti-OLLAS antibodies were detected by anti-mouse HRP (P0161, DAKO, 1:10,000). The western blots were developed using ECL Plus (GE Healthcare). LC–MS/MS analysis of a hydrogenosome-enriched fraction The amount of protein from discontinuous gradient fractionations were established by Bio-Rad Bradford assay (500–0006, Bio-Rad) using the microscale procedure in a microtitre plate. A dilution series of BSA was used to establish a standard curve. All samples and the standards were measured in triplicate in each experiment. Fifteen micrograms of proteins from fractions N1, N3 and P50 were removed for trypsin digestion. SDS and ammonium bicarbonate were added to the samples to 1% and 100 mM, respectively, and reduction and alkylation were performed with 10 mM DTT at 58 °C for 10 min followed by 20 mM iodoacetamide for 30 min in the dark at room temperature. Samples were transferred to spin tubes (Pall Corporation, 3 kDa cutoff value) for ‘filter-aided sample preparation’ [39] and urea was added to 4 M. Four exchanges with at least 10 × dilution each time was then executed and the retained volumes were estimated with a pipette. Two volumes of 100 mM ammonium bicarbonate was added and finally also CaCl 2 to 1 mM. To this, 0.5 μg Trypsin (Roche seq grade) was pipetted and digestion was allowed to proceed overnight at room temperature. The digests were made 5% in acetic acid and collected by centrifugation. The tubes were washed with 100 μL of 4 M urea/5% acetic acid, which, after centrifugation, were added to the primary filtrate. The filtrates were passed through STAGE-tips [40] two times, eluted and dried. Resolubilization was with 20 μl 0.1% trifluoroacetic acid (TFA). Mass analysis was done on a Thermo LTQ Ultra coupled with an Agilent nanoflow 1,100 HPLC. The gradient was: 2–4% B 0–10 min flow 0.5 μl min −1 , 4–35% B 10–80 min flow 0.2 μl min −1 , 35–50% B 80–98 min flow 0.2 μl min −1 , 50–100% B 98–103 min, 100% B 103–124 min flow ramped up to 0.5 μl min −1 . The column was in-house made with Repro-Sil_Pur C18AQ 3 μm beads in a fused silica capillary ~120 × 0.3 mm. The mass spectrometer was run in ft-mode with resolution 50,000, for survey scans with fragmentation in the ion-trap, which operated in a data-dependent mode. The three most abundant peptides were selected and thereafter excluded for 150 s. The resulting RAW file from the ms was converted to mgf-format by MSConvert in the ProteoWizard program suite. The FASTA file of 8067 complete genes annotated in the current version (23 April 2013) of Spironucleus salmonicida annotation were used to build the database for MASCOT [20] searches. The search parameters were set as 10 p.p.m. mass tolerance and 0.6 Da fragment mass tolerance with one missed cleavage allowed. Carbimidomethylation of cysteine was set as a fixed modification and oxidation of methionine as a variable modification. The search queries (2,474 spectra—N1 fraction; 7,046 spectra—N3 fraction; 4,760 spectra—P50 fraction) were matched to 866, 2,973 and 2,093 peptides, respectively. The peptides recovered hits to 386 proteins for the N1 fraction, 803 proteins for the N3 fraction and 744 proteins for the P50 fraction ( Supplementary Data 1 ) above the significance threshold ( P <0.05). Decoy database searches recovered 33, 143 and 88 peptide hits, indicating a false discovery rate of 3.81, 4.81 and 4.20%, respectively, for the data sets. The number of individual peptides and spectra matching proteins (expect <0.1) in the S. salmonicida hydrogenosome were extracted manually ( Supplementary Table S1 ). Supplementary Data 1 contains lists of all identified proteins in the three fractions as well as fraction unique proteins. The mass, score, queries matched and emPAI values were extracted from MASCOT HTML output with a Python script. Additional information in Supplementary Data 1 was extracted from the current annotation. Signal peptides were predicted by SignalP v4.0b (ref. 41 ); Transmembrane domains were predicted using TMHMM v2.0 (ref. 42 ); Information of the first three best Pfam (v25.0) [43] domains hits by HMMER 3.0 (ref. 44 ) were included in the table; KO and pathway were predicted by Kyoto Encyclopedia of Genes and Genomes Automatic Annotation Server [45] . Raw data from the LC–MS/MS experiment can be found at http://webdav.swegrid.se/snic/bils/uu_scilife/pub/ in the file Jerlstrom-Hultqvist_ etal _Nat_Commun_2013.zip. Accession codes: S. salmonicida nucleotide sequences for the studied genes have been deposited in Genbank/EMBL/DDBJ under accession numbers JX549066 – JX549112 and KC952876 – KC952886 . Trepomonas sp. PC1 nucleotide sequences for the studied genes have been deposited in Genbank/EMBL/DDBJ under accession numbers KF534688 – KF534705 . How to cite this article: Jerlström-Hultqvist, J. et al . Hydrogenosomes in the diplomonad Spironucleus salmonicida . Nat. Commun. 4:2493 doi: 10.1038/ncomms3493 (2013).